RETRACTED ARTICLE: SARI inhibits angiogenesis and tumour growth of human colon cancer through directly targeting ceruloplasmin SARI, also called as BATF2, belongs to the BATF family and has been implicated in cancer cell growth inhibition. However, the role and mechanism of SARI in tumour angiogenesis are elusive. Here we demonstrate that SARI deficiency facilitates AOM/DSS-induced colonic tumorigenesis in mice. We show that SARI is a novel inhibitor of colon tumour growth and angiogenesis in mice. Antibody array and HUVEC-related assays indicate that VEGF has an essential role in SARI-controlled inhibition of angiogenesis. Furthermore, Co-IP/PAGE/mass spectrometry indicates that SARI directly targets ceruloplasmin (Cp), and induces protease degradation of Cp, thereby inhibiting the activity of the HIF-1α/VEGF axis. Tissue microarray results indicate that SARI expression inversely correlates with poor clinical outcomes in colon cancer patients. Collectively, our results indicate that SARI is a potential target for therapy by inhibiting angiogenesis through the reduction of VEGF expression and is a prognostic indicator for patients with colon cancer. Colorectal cancer (CRC) is the third most common cancer in both men and women in America [1] . Surgery may be an effective way to control colorectal tumour growth at the early stage [2] , [3] , but patients are often diagnosed at an advanced stage, thereby having poor prognosis [4] . Meanwhile, targeted therapies plus cytotoxic chemotherapy has shown promising benefits in several tumour types [5] , [6] . However, targeted therapies currently face the challenge of being translated to the adjuvant setting of CRC [7] , [8] . Therefore, novel prognostic biomarkers and targeted therapeutics for CRC are needed. Basic leucine zipper (bZIP) transcription factor, ATF-like (BATF; also known as SFA2), BATF2 (also known as SARI, suppressor of activator protein 1 (AP-1), regulated by IFN) and BATF3 (also known as JDP1 and p21SNFT) comprise the BATF family [9] . It is a subgroup of the larger family of bZIP transcription factors and belongs to the AP-1 family of transcription factors, which regulate numerous cellular processes [10] . Initially, BATF family members were thought to function only as inhibitors of AP-1-driven transcription [11] , [12] ; however, recent studies have uncovered that these factors have unique, non-redundant and positive transcriptional activities in dendritic cells, B cells and T cells [13] , [14] . Thus, BATF family members are considered as attractive targets for therapy and as prognostic indicators. The SARI gene is located on human chromosome 11q (mouse chromosome 19), and the SARI protein is 47% homologous to BATF, with 59% conservation between mice and humans [9] . Recent studies have shown that SARI is downregulated in various types of cancers, and induces apoptosis in tumour cells, but not in normal cells [15] . In addition, SARI also blocks the downstream cell proliferation signals produced by CCN1 through inhibiting the activity of the CCN1 promoter [16] . Dash et al . [17] also indicated that SARI is necessary for cancer-specific killing induced by MDA-7. Furthermore, the loss of SARI expression initiates epithelial–mesenchymal transition, which is visualized by repression of E-cadherin and upregulation of vimentin in lung adenocarcinoma cell lines and in clinical lung adenocarcinoma specimens [18] . Moreover, a novel study by Liu et al . indicated that SARI is a potent negative regulator of HGF/MET signalling in CRC and may serve as a prognostic tumour marker [19] . Thus, SARI is considered an attractive target for gene therapy and indictor for patient prognosis. However, the role of SARI in tumour angiogenesis is still elusive. In this study, SARI inhibited tumour angiogenesis by directly targeting Cp and inhibiting the HIF-1α/VEGF axis with important implications for colon tumour formation in azoxymethane (AOM)/dextran sodium sulfate (DSS)-induced colonic tumorigenesis and colon cancer cell subcutaneous cancer models. Moreover, we provide tissue microarray (TMA) evidence that SARI expression inversely correlates with advanced stage and positively correlates with the survival of patients with colon cancer. Here we first determine the inhibition role of SARI in angiogenesis and colon tumour growth, and the potential use of SARI in targeted therapy and its use as a prognostic indicator for patients with colon cancer. SARI deficiency promotes AOM/DSS-induced tumorigenesis To test the role of SARI in tumorigenesis, SARI −/− and SARI WT (SARI wild type) mice were used to examine the effects of SARI on AOM/DSS-induced tumorigenesis ( Fig. 1a ). Despite that colonic tumours could be detected in both SARI −/− and SARI WT mice (mainly in the distal colons; Fig. 1b ), SARI deficiency significantly facilitated the multiplicity of colonic tumours ( Fig. 1c ) and tumour burden ( Fig. 1d ). Haematoxylin and eosin (H&E) staining also indicated that more tumour area was found in the colonic tissue of SARI −/− mice ( Fig. 1e,f ). A previous study has shown that SARI has a broad expression profile, but is not expressed in most cancer cell lines [15] . To investigate the role of SARI in colon cancer further, we measured SARI messenger RNA (mRNA) and protein expression in colon cancer cell lines by PCR with reverse transcription (RT–PCR) and western blotting. The normal colon tissue was used as a positive control. The results indicated that SARI mRNA and protein expression were not detected in any colon tumour cells except for SW620 and HCT15 cells ( Supplementary Fig. 1a,b ). Therefore, we employed the gain-of-function approach to study the SARI function in SW480 and HCT116 cells. The cells were infected with lentivirus containing either empty vector (LV-Ctrl) or a vector expressing human SARI (LV-SARI), and the stable cells were selected by puromycin, designated as SW480-SARI, HCT116-SARI, SW480-control and HCT116-control. Western blotting showed that SARI was efficiently expressed in SW480-SARI and HCT116-SARI cells, but not in control cells ( Fig. 1g ). To determine whether SARI has any effect on tumour growth in vivo , 5 × 10 6 SARI and control cancer cells were injected into the flank of female wild-type (WT) BALB/c nude mice to establish a subcutaneous tumour model. SARI staining confirmed that SARI is expressed in SW480-SARI tumours, but not in control tumours ( Fig. 1h ). Our results indicated that ectopic expression of SARI significantly reduced tumour volume and weight of SW480 cells by 80.13% and 76.05%, respectively ( Fig. 1i,j ; tumour volume: control: 565.04±73.51 mm 3 versus SARI: 112.28±36.75 mm 3 ; and tumour weight: control: 0.574±0.161 g versus SARI: 0.138±0.051 g). SARI expression also reduced tumour volume and weight of HCT16 cells by 71.66% and 72.35%, respectively ( Fig. 1k,l ; tumour volume: control: 836.87±143.18 mm 3 versus SARI: 237.19±124.62 mm 3 ; and tumour weight: control: 0.724±0.202 g versus SARI: 0.214±0.147 g). In subsequent experiments, short hairpin RNAs (shRNAs) were employed to knockdown SARI expression. We designed four shRNAs targeting SARI (shSARI-182, shSARI-554, shSARI-694 and shSARI-1068), and found that shSARI-554 and shSARI-1068 markedly inhibited SARI expression in HCT15 cells ( Supplementary Fig. 1c,d ). Our results indicated that knockdown of SARI in HCT15 cells significantly induced tumour growth ( Fig. 1m,n ; tumour volume: shNC: 448.59±88.36 mm 3 versus shSARI-1068: 1262.51±175.29 mm 3 and shSARI-554: 898.27±153.82 mm 3 ; and tumour weight: shNC: 0.517±0.167 g versus shSARI-1068: 1.403±0.387 g and shSARI-1068: 0.851±0.241 g). Collectively, the in vivo data suggest that SARI functions as a tumour suppressor. 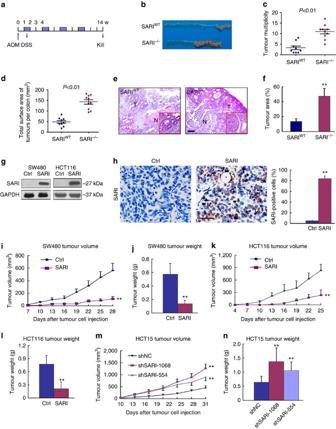Figure 1: SARI inhibits AOM/DSS-induced colonic carcinogenesis. (a) Schema of AOM/DSS treatments. (b) Representative macroscopic findings of colon tumours induced by AOM/DSS. (c,d) Number of macroscopic tumours (c) and tumour burden of AOM/DSS-treated mice (d) per colon. (SARIWT,n=9; SARI−/−,n=10;P<0.01; Student’st-test). (e,f) H&E staining of SARIWTand SARI−/−colonic tissue after AOM/DSS treatment (e). Scale bar, 100 μm. Tumour area (%, tumour area/total area) was calculated (f,n=9, **P<0.01; Student’st-test). (g) Western blot showing SARI expression in SARI and control SW480 and HCT116 cells. (h) Staining for SARI in SARI and SW480-control tumours. Scale bar, 50 μm. (i,j) Tumour volume (n=5; **P<0.01; Student’st-test) and end-stage tumour weight (n=5; **P<0.01; Student’st-test) after injection of 5 × 106SARI and SW480-control cancer cells into nude mice. (k,l) Tumour volume (n=5; **P<0.01; Student’st-test) and end-stage tumour weight (n=5; **P<0.01; Student’st-test) after injection of 5 × 106SARI and control HCT116 cancer cells into nude mice. (m,n) Tumour volume (n=5; **P<0.01; Student’sttest), and end-stage tumour weight (n=5; **P<0.01; Student’st-test) after injection of 2 × 106shSARI-1068 and shNC HCT15 cancer cells into nude mice. Ctrl, control. Figure 1: SARI inhibits AOM/DSS-induced colonic carcinogenesis. ( a ) Schema of AOM/DSS treatments. ( b ) Representative macroscopic findings of colon tumours induced by AOM/DSS. ( c , d ) Number of macroscopic tumours ( c ) and tumour burden of AOM/DSS-treated mice ( d ) per colon. (SARI WT , n =9; SARI −/− , n =10; P <0.01; Student’s t -test). ( e , f ) H&E staining of SARI WT and SARI −/− colonic tissue after AOM/DSS treatment ( e ). Scale bar, 100 μm. Tumour area (%, tumour area/total area) was calculated ( f , n =9, ** P <0.01; Student’s t -test). ( g ) Western blot showing SARI expression in SARI and control SW480 and HCT116 cells. ( h ) Staining for SARI in SARI and SW480-control tumours. Scale bar, 50 μm. ( i , j ) Tumour volume ( n =5; ** P <0.01; Student’s t -test) and end-stage tumour weight ( n =5; ** P <0.01; Student’s t -test) after injection of 5 × 10 6 SARI and SW480-control cancer cells into nude mice. ( k , l ) Tumour volume ( n =5; ** P <0.01; Student’s t -test) and end-stage tumour weight ( n =5; ** P <0.01; Student’s t -test) after injection of 5 × 10 6 SARI and control HCT116 cancer cells into nude mice. ( m , n ) Tumour volume ( n =5; ** P <0.01; Student’s t test), and end-stage tumour weight ( n =5; ** P <0.01; Student’s t -test) after injection of 2 × 10 6 shSARI-1068 and shNC HCT15 cancer cells into nude mice. Ctrl, control. Full size image SARI inhibits angiogenesis in vivo and in vitro We next stained the tumours with CD31 antibody, which recognizes endothelial cells, to observe angiogenesis. The results showed that vessel density and average vessel area were lower in SW480-SARI tumours than in control tumours ( Fig. 2a–c ). Meanwhile, more vessels were found in HCT15 tumours after knockdown of SARI, compared with the shNC group ( Supplementary Fig. 2a ). Since blockage of angiogenesis often induces tumour necrosis and hypoxia, we employed H&E and pimonidazole (PIMO) staining to examine the effects of SARI on these factors. H&E staining showed that SARI induces necrosis in SW480 tumours ( Fig. 2d,e ). Consistently, PIMO staining indicated that SW480-SARI tumours were more hypoxic than control tumours ( Fig. 2f,g ). Moreover, staining for an apoptosis marker (cleaved caspase-3 combined with CD31) showed that blockage of angiogenesis by SARI induces apoptosis in SW480 tumour ( Fig. 2h,i ). In addition, there was an inverse correlation between cleaved caspase-3 and CD31. It is indicated that the apoptosis of SW480 tumours is a result of the blockage of angiogenesis, but not the direct result of SARI. Similar results also were found in HCT116-SARI and HCT116-comtrol tumours ( Supplementary Fig. 2b–e ). Taken together, our results suggest that overexpression of SARI in colon cancer cells significantly inhibits tumour growth in vivo through the inhibition of angiogenesis. 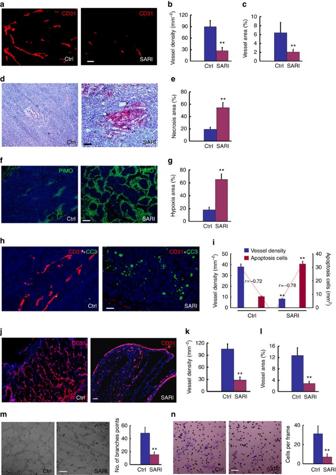Figure 2: SARI inhibits angiogenesisin vivoandin vitro. (a–c) Staining for CD31 (red) in control and SARI SW480 tumours. Vessel density (b; mm−2;n=5; **P<0.01; Student’st-test) and vessel area (c; %;n=5; **P<0.01; Student’st-test) were quantified. Scale bar, 100 μm. (d,e) H&E staining for SARI and control SW480 tumours after tumour cell injection for 25 days (d). Analysis of necrotic area (e, % of tumour area;n=5; **P<0.01; Student’st-test). Scale bar, 100 μm. (f,g) Staining for pimonidazole (PIMO; green) in SARI and SW480-control tumours (f). Analysis of PIMO area (% of tumour area;g,n=5; **P<0.01; Student’st-test). DAPI staining for the nucleus. Scale bar, 100 μm. (h,i) Staining for cleaved caspase-3 (green, CC3) and CD31 (red) in SARI and control SW480 tumours (h); apoptotic cells and vessel density were counted (i,n=5; **P<0.01; Student’st-test). The correlation between CC3 and CD31 was analysed, and the red line indicates the correlation (Pearson correlation analysis). DAPI staining for the nucleus. Scale bar, 50 μm. (j–l) Staining for CD31 (red) in control and SARISW480 Matrigel plugs (j) revealed that SARI inhibits angiogenesis in SW480-matrigel plugs. Vessel density (k; mm−2;n=5; **P<0.01; Student’st-test) and vessel area (l; %;n=5; **P<0.01; Student’st-test) were quantified. Scale bar, 100 μm. (m) Endothelial tube formation was estimated following incubation of HUVECs with conditioned medium from SW480-control and SARI cancer cells. The number of branches were quantified (n=5; **P<0.01; Student’st-test). Scale bar, 50 μm. (n) Representative photomicrographs of HUVECs that have invaded through Matrigel chambers after incubation with conditioned medium from SW480-control and SARI cancer cells for 72 h. Scale bar, 50 μm. Quantification of HUVECs that have invaded through Matrigel chambers (n=5; **P<0.01; Student’st-test). Ctrl, control. Figure 2: SARI inhibits angiogenesis in vivo and in vitro . ( a – c ) Staining for CD31 (red) in control and SARI SW480 tumours. Vessel density ( b ; mm −2 ; n =5; ** P <0.01; Student’s t -test) and vessel area ( c ; %; n =5; ** P <0.01; Student’s t -test) were quantified. Scale bar, 100 μm. ( d , e ) H&E staining for SARI and control SW480 tumours after tumour cell injection for 25 days ( d ). Analysis of necrotic area ( e , % of tumour area; n =5; ** P <0.01; Student’s t -test). Scale bar, 100 μm. ( f , g ) Staining for pimonidazole (PIMO; green) in SARI and SW480-control tumours ( f ). Analysis of PIMO area (% of tumour area; g , n =5; ** P <0.01; Student’s t -test). DAPI staining for the nucleus. Scale bar, 100 μm. ( h , i ) Staining for cleaved caspase-3 (green, CC3) and CD31 (red) in SARI and control SW480 tumours ( h ); apoptotic cells and vessel density were counted ( i , n =5; ** P <0.01; Student’s t -test). The correlation between CC3 and CD31 was analysed, and the red line indicates the correlation (Pearson correlation analysis). DAPI staining for the nucleus. Scale bar, 50 μm. ( j – l ) Staining for CD31 (red) in control and SARISW480 Matrigel plugs ( j ) revealed that SARI inhibits angiogenesis in SW480-matrigel plugs. Vessel density ( k ; mm −2 ; n =5; ** P <0.01; Student’s t -test) and vessel area ( l ; %; n =5; ** P <0.01; Student’s t -test) were quantified. Scale bar, 100 μm. ( m ) Endothelial tube formation was estimated following incubation of HUVECs with conditioned medium from SW480-control and SARI cancer cells. The number of branches were quantified ( n =5; ** P <0.01; Student’s t -test). Scale bar, 50 μm. ( n ) Representative photomicrographs of HUVECs that have invaded through Matrigel chambers after incubation with conditioned medium from SW480-control and SARI cancer cells for 72 h. Scale bar, 50 μm. Quantification of HUVECs that have invaded through Matrigel chambers ( n =5; ** P <0.01; Student’s t -test). Ctrl, control. Full size image To verify the effects of SARI on angiogenesis in vivo further, a Matrigel plug assay was performed following subcutaneous injection of Matrigel-loaded colon cancer cells in BALB/c nude mice. Staining for CD31 showed that vessel density and average vessel area were lower in SW480-SARI tumours than in control tumours ( Fig. 2j–l ). To determine the effect of SARI on angiogenesis in vitro , conditional medium after 48 h of culture was used for human umbilical vein endothelial cell (HUVEC) tube formation and invasion assays. The results showed that there are fewer branch points in the conditional medium from SW480-SARI cells than that from SW480-control cells ( Fig. 2m ). Meanwhile, a lower invasion rate was also found in HUVECs treated with SW480-SARI conditional medium than in those treated with the control medium ( Fig. 2n ). Collectively, our results further demonstrate the role of SARI in inhibiting angiogenesis in colon cancer. VEGF mediates angiogenesis inhibition of SARI controlled An angiogenesis antibody array was performed to determine the difference in expression angiogenesis-related cytokines between the conditional medium of SW480-cotrol and SW480-SARI cells. The results in Fig. 3a,b show that levels of five cytokines, EGF, bFGF, PDGF-BB, PLGF and VEGF, decreased in SW480-SARI supernatant compared with those of the SW480-control group. Enzyme-linked immunosorbent assay (ELISA) further confirmed that VEGF expression was significantly inhibited by SARI in both SW480 and HCT116 cells ( Fig. 3c ). Meanwhile, reduction of other cytokines by SARI has been demonstrated by ELISA ( Supplementary Fig. 3a ). Western blotting showed similar results ( Fig. 3d ). Moreover, immunofluorescence analysis confirmed that VEGF expression was reduced in both SW480 and HCT116 cells with the stable expression of SARI ( Fig. 3e ). VEGF mRNA expression was determined by real-time PCR and the results indicated that SARI inhibits the expression of VEGF at a transcriptional level ( Supplementary Fig. 3b ). For additional experiments, a doxycycline-based inducible expression plasmid was constructed. After treatment with doxycycline (20 μg ml −1 ) for 48 h, high expression of SARI was observed in the pLVX-Tet-SARI-transfected cells ( Supplementary Fig. 3c ). Meanwhile, accompanied with high expression of SARI, a reduction in VEGF expression was observed ( Supplementary Fig. 3c ). Inhibition of SARI by shSARI-554 and shSARI-1068 in HCT15 and SW620 cells also caused significant upregulation of VEGF expression ( Supplementary Fig. 3d ). Since SARI inhibits HUVEC tube formation and invasion, we questioned whether VEGF-mediated angiogenesis inhibition was SARI controlled. Hence, shRNAs were employed to knockdown VEGF expression. We designed four shRNAs targeting VEGF (shVEGF-1060, shVEGF-1172, shVEGF-442 and shVEGF-901), and found that shVEGF-442 and shVEGF-901 were able to inhibit VEGF expression in SW480 cells markedly ( Supplementary Fig. 3e ). HUVEC tube formation ( Fig. 3f,g ) and invasion assays ( Fig. 3h,i ) suggested that there were no significant differences between Ctrl and SARI groups after knockdown of VEGF. Furthermore, recombinant VEGF protein and VEGF-neutralizing antibody, VEGF-trap, were also used to increase or inhibit VEGF expression, respectively. The results showed that the addition of recombinant VEGF protein significantly increased HUVEC tube formation and invasion, whereas no significant differences were observed between the Ctrl+VT and the SARI+VT groups ( Supplementary Fig. 3f,g ). Therefore, VEGF is the molecular target of SARI during angiogenesis inhibition. 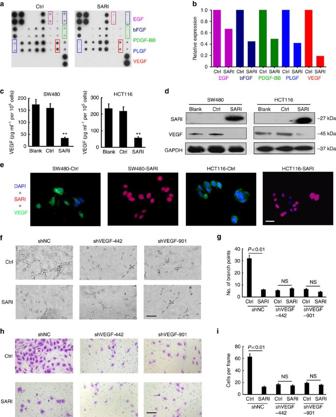Figure 3: Reduction of VEGF by SARI. (a) Human angiogenesis array analysis of the conditional medium from SW480-controland SW480-SARI cells. (b) Summary of the relative signal intensity of indicated cytokines. (c) VEGF exacted from SW480 and HCT116 cells was quantified by ELISA (n=3; **P<0.01; Student’st-test). (d) Western blot showing expression of the SARI protein and that SARI inhibits cellular VEGF expression in SW480 and HCT116 cellsin vitro. (e) Staining for SARI (red) and VEGF (green) in SW480-control, SW480-SARI, HCT116-control and HCT116-SARI cells; DAPI staining for the nucleus. Scale bar, 50 μm. (f,g) Endothelial tube formation estimation following the incubation of HUVECs with conditioned medium from SW480-control, SW480-SARIcancer cells with or without shVEGF-442, or shVEGF-901 transfection. The number of branches was quantified (g;n=5;P<0.01; NS, no significant difference; Student’st-test). Scale bar, 50 μm. (h,i) Representative photomicrographs of HUVECs that have invaded through Matrigel chambers after incubation with conditioned medium for 72 h from SW480-control, SW480-SARI cancer cells with or without shVEGF-442, or shVEGF-901 transfection. Scale bar, 50 μm. (i) Quantification of HUVECs that have invaded through Matrigel chambers (n=5;P<0.01; NS, no significant difference; Student’st-test). Ctrl, control. Figure 3: Reduction of VEGF by SARI. ( a ) Human angiogenesis array analysis of the conditional medium from SW480-controland SW480-SARI cells. ( b ) Summary of the relative signal intensity of indicated cytokines. ( c ) VEGF exacted from SW480 and HCT116 cells was quantified by ELISA ( n =3; ** P <0.01; Student’s t -test). ( d ) Western blot showing expression of the SARI protein and that SARI inhibits cellular VEGF expression in SW480 and HCT116 cells in vitro . ( e ) Staining for SARI (red) and VEGF (green) in SW480-control, SW480-SARI, HCT116-control and HCT116-SARI cells; DAPI staining for the nucleus. Scale bar, 50 μm. ( f , g ) Endothelial tube formation estimation following the incubation of HUVECs with conditioned medium from SW480-control, SW480-SARIcancer cells with or without shVEGF-442, or shVEGF-901 transfection. The number of branches was quantified ( g ; n =5; P <0.01; NS, no significant difference; Student’s t -test). Scale bar, 50 μm. ( h , i ) Representative photomicrographs of HUVECs that have invaded through Matrigel chambers after incubation with conditioned medium for 72 h from SW480-control, SW480-SARI cancer cells with or without shVEGF-442, or shVEGF-901 transfection. Scale bar, 50 μm. ( i ) Quantification of HUVECs that have invaded through Matrigel chambers ( n =5; P <0.01; NS, no significant difference; Student’s t -test). Ctrl, control. Full size image SARI reduces VEGF expression by directly targeting Cp Further, to determine the direct target of SARI in the regulation of VEGF expression, co-immunoprecipitation (Co-IP) and mass spectrometry (MS) were performed. SW480-control and SW480-SARI cell proteins were collected, and anti-SARI antibody was added to pull down the SARI and direct target protein. The products were separated by SDS–polyacrylamide gel electrophoresis (SDS–PAGE) and the unique band was subjected to MS analysis. As shown in Fig. 4a , ceruloplasmin (Cp) was predicted as the direct target of SARI. To determine the distribution of Cp, the normal human colonic epithelial cell line, HCoEpiC and colon cancer cell line were employed for Cp staining. The results indicated that Cp localized in the cytoplasm of HCoEpiC cells, whereas it localized in the nucleus of human colon cancer cells ( Supplementary Fig. 4a ). Furthermore, malignant colonic tissues and adjacent normal colonic tissues from patients were collected and used for Cp staining. It is indicated that Cp localized in the cytoplasm of normal colonic tissues, whereas Cp mostly localized in the nucleus of malignant colonic tissues ( Supplementary Fig. 4b ). Then, we collected SW480-control and SW480-SARI cells, and performed immunoprecipitation. Western blotting showed that SARI and Cp reciprocally interact with one another ( Fig. 4b ). Further immunofluorescence analysis revealed that SARI (red) and Cp (green) were co-localized in the nucleus (4,6-diamidino-2-phenylindole (DAPI) staining; Fig. 4c ). It was indicated that Cp directly interacted with SARI. Notably, western blotting showed that SARI significantly inhibited Cp expression in both SW480 and HCT116 cells ( Fig. 4d ). Cp mRNA expression was determined by real-time PCR and there was no significant difference between the control and SARI groups for both SW480 and HCT116 cells ( Supplementary Fig. 5a ). Nuclear and cytoplasmic proteins of SW480-control and SW480-SARI cells were collected and used for western blotting. The results indicated that SARI inhibited nuclear Cp expression, but cytoplasmic ( Fig. 4e ). After treatment with MG132, a specific proteasome inhibitor, SARI-induced reduction of Cp and VEGF expression was blocked ( Fig. 4f,g ). To measure the kinetics of Cp protein degradation, we added cycloheximide to arrest protein synthesis. The degradation rate of existing Cp protein was obtained by measuring Cp levels in cell lysates harvested at 0, 2, 4, 6, 8 and 10 h after cycloheximide addition. We observed that the Cp protein was degraded faster in the SARI cells than in the control cells ( Fig. 4h ), which was confirmed by densitometry of multiple western blotting analysis results ( Fig. 4i ). Moreover, inhibition of SARI expression by shRNA upregulated the expression of Cp in HCT15 cells ( Fig. 4j ). These results indicated that SARI directly target Cp, and hence inhibits the expression of Cp using the protein degradation pathway. Stepwise deletion of SARI indicated that amino acids 80–274 bear the role of reducing Cp expression ( Fig. 4k ). Co-IP results also indicated that the binding site of Cp is localized among amino acids 80–274 of SARI ( Fig. 4l ), but the exact binding site should be determined in further studies. If the interaction is disrupted, the inhibition of VEGF expression ( Fig. 4m ) and the subsequent HUVEC tube formation ( Supplementary Fig. 5b ) controlled by SARI disappeared. 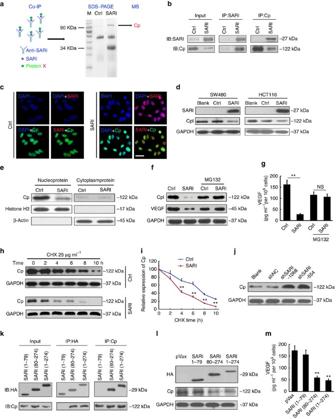Figure 4: SARI inhibits VEGF expression by directly binding to Cp. (a) Co-immunoprecipitation products after adding anti-SARI antibody were separated by SDS–PAGE, and the differential band was analysed by MS. (b) Co-immunoprecipitation analysis of SW480-control and SW480-SARI cell lysates using anti-SARI and anti-Cp antibody. (c) Staining for Cp (green) and SARI (red) in SW480-control and SW480-SARI cells; DAPI staining for the nucleus. Scale bar, 50 μm. (d) Immunoblots of SARI and Cp expression in SW480 and HCT116-blank, control and SARI cells. GAPDH was used as a loading control. (e) Western blotting detection of Cp expression of collected nuclear and cytoplasmic proteins. Histone H3 was used as the nucleus loading control and β-actin as the cytoplasm loading control. (f) Immunoblots of Cp and VEGF expression in SW480-control and SW480-SARI cells with or without MG132 treatment. GAPDH was used as the loading control. (g) ELISA detection of VEGF expression in SW480-control and SW480-SARI cells with or without MG132 treatment. (n=4; **P<0.01; Student’st-test) (h) Measurement of Cp in cell lysates harvested at 0, 2, 4, 6, 8 and 10 h after the addition of cycloheximide (CHX) to arrest protein synthesis. (i) Densitometry analysis of Cp expression in multiple western blots after CHD addition (n=3; **P<0.01; Student’st-test). (j) Immunoblots of Cp expression in HCT15, HCT15-shNC, HCT15-shSARI-1068 and HCT15-shSARI-554 cells. GAPDH was used as a loading control. (k) Co-immunoprecipitation analysis using anti-HA and anti-CP antibodies of total cell lysates collected from SW480 cells after transfection with HA-SARI (encoding 1–79 amino acids), HA-SARI (encoding 80–274 amino acids) and HA-SARI (encoding 1–274 amino acids). Immunoblots of HA and Cp expression. (l) Immunoblots of HA and Cp expression in SW480 cells after transfection with pVax, HA-SARI (encoding 1–79 amino acids), HA-SARI (encoding 80–274 amino acids) and HA-SARI (encoding 1–274 amino acids). GAPDH was used as a loading control. (m) ELISA detection of VEGF expression in the conditional medium from the SW480 cells after transfection with pVax, HA-SARI (encoding 1–79 amino acids), HA-SARI (encoding 80–274 amino acids) and HA-SARI (encoding 1–274 amino acids) with or without TM (4.0 μM) treatment. (n=3; **P<0.01; analysis of variance analysis). IB, immuoblot. Figure 4: SARI inhibits VEGF expression by directly binding to Cp. ( a ) Co-immunoprecipitation products after adding anti-SARI antibody were separated by SDS–PAGE, and the differential band was analysed by MS. ( b ) Co-immunoprecipitation analysis of SW480-control and SW480-SARI cell lysates using anti-SARI and anti-Cp antibody. ( c ) Staining for Cp (green) and SARI (red) in SW480-control and SW480-SARI cells; DAPI staining for the nucleus. Scale bar, 50 μm. ( d ) Immunoblots of SARI and Cp expression in SW480 and HCT116-blank, control and SARI cells. GAPDH was used as a loading control. ( e ) Western blotting detection of Cp expression of collected nuclear and cytoplasmic proteins. Histone H3 was used as the nucleus loading control and β-actin as the cytoplasm loading control. ( f ) Immunoblots of Cp and VEGF expression in SW480-control and SW480-SARI cells with or without MG132 treatment. GAPDH was used as the loading control. ( g ) ELISA detection of VEGF expression in SW480-control and SW480-SARI cells with or without MG132 treatment. ( n =4; ** P <0.01; Student’s t -test) ( h ) Measurement of Cp in cell lysates harvested at 0, 2, 4, 6, 8 and 10 h after the addition of cycloheximide (CHX) to arrest protein synthesis. ( i ) Densitometry analysis of Cp expression in multiple western blots after CHD addition ( n =3; ** P <0.01; Student’s t -test). ( j ) Immunoblots of Cp expression in HCT15, HCT15-shNC, HCT15-shSARI-1068 and HCT15-shSARI-554 cells. GAPDH was used as a loading control. ( k ) Co-immunoprecipitation analysis using anti-HA and anti-CP antibodies of total cell lysates collected from SW480 cells after transfection with HA-SARI (encoding 1–79 amino acids), HA-SARI (encoding 80–274 amino acids) and HA-SARI (encoding 1–274 amino acids). Immunoblots of HA and Cp expression. ( l ) Immunoblots of HA and Cp expression in SW480 cells after transfection with pVax, HA-SARI (encoding 1–79 amino acids), HA-SARI (encoding 80–274 amino acids) and HA-SARI (encoding 1–274 amino acids). GAPDH was used as a loading control. ( m ) ELISA detection of VEGF expression in the conditional medium from the SW480 cells after transfection with pVax, HA-SARI (encoding 1–79 amino acids), HA-SARI (encoding 80–274 amino acids) and HA-SARI (encoding 1–274 amino acids) with or without TM (4.0 μM) treatment. ( n =3; ** P <0.01; analysis of variance analysis). IB, immuoblot. Full size image SARI inhibits the activity of the HIF-1α/VEGF axis Previous studies indicated that HIF-1α is one of the downstream targets of Cp [20] . Thus, we examined HIF-1α expression in SW480-control and SW480-SARI cells. We found SARI significantly inhibits the expression of HIF-1α ( Fig. 5a ). To compensate for the low expression of HIF-1α protein seen in HCT116 cells ( Supplementary Fig. 6a ), we treated HCT116 cells with 1% O 2 and dimethyloxalylglycine (DMOG), an inhibitor of HIF-1α degradation, to induce HIF-1α expression ( Supplementary Fig. 6b,c ). Results demonstrated that HIF-1α expression was also reduced by SARI in HCT116 cells after treatment with 1% O 2 and DMOG ( Fig. 5a ). To further confirm that Cp regulates SARI inhibition of HIF-1α, PX-478, a specific inhibitor of HIF-1α ( Supplementary Fig. 6d ), and tetrathiomolybdate (Tm), a specific inhibitor of Cp ( Supplementary Fig. 6e ), were used. Cp and HIF-1α expression was significantly inhibited by Tm in a concentration-dependent manner ( Supplementary Fig. 5e ). PX-478 and Tm treatment blocked the SARI-controlled inhibition of Cp, HIF-1α and VEGF expression in normoxic and hypoxia conditions ( Fig. 5b ). After overexpression of Cp, the SARI-controlled inhibition on HIF-1α expression was also blocked in normoxic and hypoxia conditions ( Fig. 5c ). ELISA detection of VEGF was consistent with the above findings ( Fig. 5d ). Moreover, HUVEC tube formation and invasion assays were performed to assess this possibility. As shown in Fig. 5e,f , the condition medium from SW480-SARI cells markedly inhibited both HUVEC tube formation and invasion. Meanwhile, there was no significant difference between SW480-control and SW480-SARI cells on either of these events after inhibition or overexpression of Cp in cells ( Fig. 5e,f ). Furthermore, Tm was demonstrated to block the upregulation of HIF-1α and VEGF expression by shSARI-1068 and shSARI-554 ( Fig, 5g,h ). The conditioned medium from HCT15-shSARI-1068 or HCT15-shSARI-554 cells significantly induced HUVEC tube formation and invasion compared with that from HCT15 cells ( Supplementary Fig. 6f,g ). However, the effects were also blocked after inhibition of Cp expression in the cells ( Supplementary Fig. 6f,g ). All the above results indicated that SARI inhibits VEGF expression and angiogenesis through directly targeting Cp and hence inhibits the activity of the HIF-1α/VEGF axis. 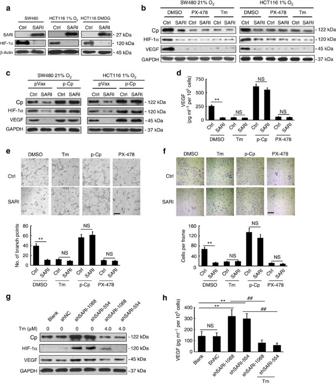Figure 5: SARI inhibits angiogenesis through inhibiting Cp expression and the activity of the HIF-1α/VEGF axis. (a) Immunoblots of SARI and HIF-1α expression in SW480 and HCT116 cells after stable expression of SARI. HCT116-control and HCT116-SARI cells were incubated under 1% O2for 48 h or treated with DMOG for 24 h. β-Actin was used as a loading control. (b) Immunoblots of Cp, HIF-1α and VEGF expression in control and SARI cells with or without PX-478 (45 μM) or Tm (4.0 μM) treatment under normoxia and hypoxia. GAPDH was used as the loading control. (c) Immunoblots of Cp, HIF-1α and VEGF expression in control and SARI cells after transfection with or without p-Cp plasmid under normoxia and hypoxia. GAPDH was used as the loading control. (d) Expression of VEGF exacted by SW480-control and SW480-SARI cells with or without Tm (4.0 μM) and PX-478 (45 μM) treatment, after transfection with or without Cp expression plasmid (n=3; **P<0.01, NS, no significant difference; Student’st-test). (e) Endothelial tube formation estimation following the incubation of HUVECs with conditioned medium from SW480-control and SW480-SARI cells with or without Tm treatment (4.0 μM) and PX-478 (45 μM), after transfection with or without Cp expression plasmid. The number of branches were quantified (n=5; **P<0.01; NS, no significant difference; Student’st-test). Scale bar, 50 μm. (f) Representative photomicrographs of HUVECs that have invaded through Matrigel chambers after incubation with conditioned medium from SW480-control and SW480-SARI cells with or without Tm treatment (4.0 μM) and PX-478 (45 μM), after transfection with or without Cp expression plasmid. Quantification of HUVECs that have invaded through Matrigel chambers (n=5; **P<0.01; NS, no significant difference; Student’st-test). (g) Immunoblots of Cp and HIF-1α expression in HCT15, HCT15-shNC, HCT15-shSARI-1068 and HCT15-shSARI-554 cells with or without Tm (4.0 μM) treatment. GAPDH was used as a loading control. (h) Expression of VEGF exacted by HCT15, HCT15-shNC, HCT15-shSARI-1068 and HCT15-shSARI-554 cells with or without Tm treatment (4.0 μM) was measured by ELISA (n=3; **P<0.01;##P<0.01; analysis of variance analysis). Figure 5: SARI inhibits angiogenesis through inhibiting Cp expression and the activity of the HIF-1α/VEGF axis. ( a ) Immunoblots of SARI and HIF-1α expression in SW480 and HCT116 cells after stable expression of SARI. HCT116-control and HCT116-SARI cells were incubated under 1% O 2 for 48 h or treated with DMOG for 24 h. β-Actin was used as a loading control. ( b ) Immunoblots of Cp, HIF-1α and VEGF expression in control and SARI cells with or without PX-478 (45 μM) or Tm (4.0 μM) treatment under normoxia and hypoxia. GAPDH was used as the loading control. ( c ) Immunoblots of Cp, HIF-1α and VEGF expression in control and SARI cells after transfection with or without p-Cp plasmid under normoxia and hypoxia. GAPDH was used as the loading control. ( d ) Expression of VEGF exacted by SW480-control and SW480-SARI cells with or without Tm (4.0 μM) and PX-478 (45 μM) treatment, after transfection with or without Cp expression plasmid ( n =3; ** P <0.01, NS, no significant difference; Student’s t -test). ( e ) Endothelial tube formation estimation following the incubation of HUVECs with conditioned medium from SW480-control and SW480-SARI cells with or without Tm treatment (4.0 μM) and PX-478 (45 μM), after transfection with or without Cp expression plasmid. The number of branches were quantified ( n =5; ** P <0.01; NS, no significant difference; Student’s t -test). Scale bar, 50 μm. ( f ) Representative photomicrographs of HUVECs that have invaded through Matrigel chambers after incubation with conditioned medium from SW480-control and SW480-SARI cells with or without Tm treatment (4.0 μM) and PX-478 (45 μM), after transfection with or without Cp expression plasmid. Quantification of HUVECs that have invaded through Matrigel chambers ( n =5; ** P <0.01; NS, no significant difference; Student’s t -test). ( g ) Immunoblots of Cp and HIF-1α expression in HCT15, HCT15-shNC, HCT15-shSARI-1068 and HCT15-shSARI-554 cells with or without Tm (4.0 μM) treatment. GAPDH was used as a loading control. ( h ) Expression of VEGF exacted by HCT15, HCT15-shNC, HCT15-shSARI-1068 and HCT15-shSARI-554 cells with or without Tm treatment (4.0 μM) was measured by ELISA ( n =3; ** P <0.01; ## P <0.01; analysis of variance analysis). Full size image SARI inhibits angiogenesis and VEGF expression in vivo The above results indicated that SARI inhibits angiogenesis through inactivation of the HIF-1α/VEGF axis. To verify the mechanism, we determined the expression of related molecules by immunostaining and immunofluorescence. We found that overexpression of SARI in SW480 cells significantly inhibited VEGF expression both in Matrigel plug tumours ( Fig. 6a ) and in subcutaneous tumours ( Fig. 6b ). Furthermore, fewer Cp- ( Fig. 6c ) and HIF-1α-( Fig. 6d ) positive cells were found in the SW480-SARI subcutaneous tumours compared with the SW480-control group. In subsequent experiments, protein was exacted from SW480 subcutaneous tumours, and western blotting and ELISA results indicated that VEGF, Cp and HIF-1α were all inhibited by SARI ( Fig. 6e,f ). Moreover, we examined the angiogenesis of AMO/DSS-induced colonic tumours by CD31 staining ( Fig. 6g ) and the results indicated that SARI deficiency markedly promotes angiogenesis. To further confirm the signalling pathway that SARI regulates, AMO/DSS-induced colonic tumours from SARI −/− and SARI WT mice were used for VEGF, Cp and HIF-1α immunohistochemistry staining ( Fig. 6g ). The results revealed that more VEGF-, Cp- and HIF-1α-( Fig. 6g ) positive cells were found in colonic tumours from SARI −/− mice. Western blotting and ELISA detection of VEGF, Cp and HIF-1α in the proteins exacted from AMO/DSS-induced colonic tumours also confirmed these findings ( Fig. 6h,i ). Further results indicated that SARI deficiency promotes the expression of Cp in the nucleus, but not in the cytoplasm ( Fig. 6j ). These data suggest that SARI impairs AOM/DSS-induced colonic tumour formation and progression through inhibiting angiogenesis and downregulating the expression of VEGF, Cp and HIF-1α. 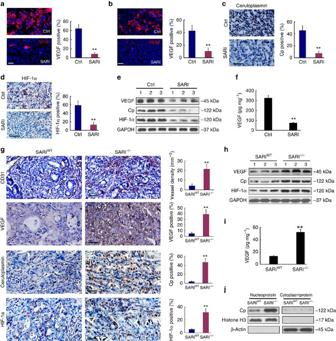Figure 6: SARI inhibits expression of downstream targetsin vivo. (a) Staining for VEGF (red) revealed less VEGF-positive cells in SARI than in controlSW480Matrigel plugs, Scale bar, 50 μm; VEGF-positive (%; VEGF positive per total cells;n=5; **P<0.01; Student’st-test). (b) Staining for VEGF (red) revealed less VEGF-positive cells in SARI than in control HCT116 tumours (d), Scale bar, 100 μm; VEGF positive (%;VEGF positive per total cells;n=5; **P<0.01; Student’st-test). (c) Staining for Cp revealed less Cp-positive cells in SARI than in control HCT116 tumours, Scale bar, 100 μm; Cp positive (%;Cp positive per total cells;n=5; **P<0.01; Student’st-test). (d) Staining for HIF-1α (red)-positive cells in SARI and control HCT116 tumours, Scale bar, 100 μm; HIF-1α positive (%; HIF-1α positive per total cells;n=5; **P<0.01; Student’st-test). (e) Immunoblots of VEGF, Cp and HIF-1a expression in SW480-control and SW480-SARI tumours. GAPDH was used as the loading control. (f) ELISA detection of VEGF expression in SW480-control and SW480-SARI tumours (n=3; **P<0.01; Student’st-test). (g) Staining for CD31, VEGF, Cp and HIF-1α in colonic tumours of AOM/DSS induction. Analysis of the number of microvessels, VEGF-positive cells, Cp-positive cells and HIF-1α-positive cells (n=4; **P<0.01; Student’st-test). Scale bar, 100 μm. (h) Immunoblots of VEGF, Cp and HIF-1α expression in colonic tumours of SARI−/−and SARIWTmice after AOM/DSS induction. GAPDH was used as the loading control. (i) ELISA detection of VEGF expression in colonic tumours of SARI−/−and SARIWTmice after AOM/DSS induction. (n=3; **P<0.01; Student’st-test) (j) Nuclear and cytoplasmic proteins were collected from the colonic tumours of SARI−/−and SARIWTmice after AOM/DSS induction. Western blotting was performed to detect Cp expression. Histone H3 was used as the nuclear loading control and β-actin as the cytoplasmic loading control. Figure 6: SARI inhibits expression of downstream targets in vivo . ( a ) Staining for VEGF (red) revealed less VEGF-positive cells in SARI than in controlSW480Matrigel plugs, Scale bar, 50 μm; VEGF-positive (%; VEGF positive per total cells; n =5; ** P <0.01; Student’s t -test). ( b ) Staining for VEGF (red) revealed less VEGF-positive cells in SARI than in control HCT116 tumours ( d ), Scale bar, 100 μm; VEGF positive (%;VEGF positive per total cells; n =5; ** P <0.01; Student’s t -test). ( c ) Staining for Cp revealed less Cp-positive cells in SARI than in control HCT116 tumours, Scale bar, 100 μm; Cp positive (%;Cp positive per total cells; n =5; ** P <0.01; Student’s t -test). ( d ) Staining for HIF-1α (red)-positive cells in SARI and control HCT116 tumours, Scale bar, 100 μm; HIF-1α positive (%; HIF-1α positive per total cells; n =5; ** P <0.01; Student’s t -test). ( e ) Immunoblots of VEGF, Cp and HIF-1a expression in SW480-control and SW480-SARI tumours. GAPDH was used as the loading control. ( f ) ELISA detection of VEGF expression in SW480-control and SW480-SARI tumours ( n =3; ** P <0.01; Student’s t -test). ( g ) Staining for CD31, VEGF, Cp and HIF-1α in colonic tumours of AOM/DSS induction. Analysis of the number of microvessels, VEGF-positive cells, Cp-positive cells and HIF-1α-positive cells ( n =4; ** P <0.01; Student’s t -test). Scale bar, 100 μm. ( h ) Immunoblots of VEGF, Cp and HIF-1α expression in colonic tumours of SARI −/− and SARI WT mice after AOM/DSS induction. GAPDH was used as the loading control. ( i ) ELISA detection of VEGF expression in colonic tumours of SARI −/− and SARI WT mice after AOM/DSS induction. ( n =3; ** P <0.01; Student’s t -test) ( j ) Nuclear and cytoplasmic proteins were collected from the colonic tumours of SARI −/− and SARI WT mice after AOM/DSS induction. Western blotting was performed to detect Cp expression. Histone H3 was used as the nuclear loading control and β-actin as the cytoplasmic loading control. Full size image SARI inversely correlates with poor prognosis of patients Further, to determine its prognostic significance in patients with colon cancer, we analysed SARI expression by immunohistochemistry staining in a cohort of 135 pairs of human malignant colon cancer tissues and their adjacent noncancerous colon tissues. Compared with normal colon tissue, SARI expression was significantly reduced in 106 (78.52%) of the 135 malignant colon cancer specimens ( Fig. 7a,b ). Furthermore, SARI expression was analysed by immunohistochemistry staining in 90 colon cancer patients at different stages, and the results showed that SARI expression inversely correlates with tumour grade ( Fig. 7c ). Most importantly, the frequency of SARI staining was positively correlated with overall survival ( Fig. 7d ). On the basis of the previous results, we hypothesized that SARI expression is associated with angiogenesis, and VEGF, Cp and HIF-1α expression in malignant colon tissues from patients with CRC. To explore this, 20 pairs of colon tissue from patients were collected and used ( Supplementary Fig. 7a ). SARI expression was determined by western blotting and immunohistochemistry ( Supplementary Fig. 7b ), and the density was measured by the Image J software ( Supplementary Fig. 7c ). CD31, VEGF, Cp and HIF-1α expression was determined by immunohistochemistry staining and scored as outlined in the methods ( Fig. 7e ). We detected a significant inverse correction between the expression of SARI and CD31 ( r =−0.633, P =0.003), SARI and VEGF ( r =−0.742, P =0.001), SARI and Cp ( r =−0.692, P =0.001), and SARI and HIF-1α ( r =−0.686, P =0.001; Fig. 7f ). These observations are consistent with the role of SARI in downregulating VEGF through the HIF-1α/VEGF axis in tumour-bearing colonic xenograft tumours. According to these findings, we hypothesize that SARI inhibits VEGF expression at the transcriptional level through the HIF-1α/VEGF axis by directly targeting Cp, hence inhibiting HIF-1α expression ( Fig. 7g ). Taken together, our results indicated that SARI is a prognostic indicator for patients with colon cancer and may play a role in tumour angiogenesis by targeting VEGF. 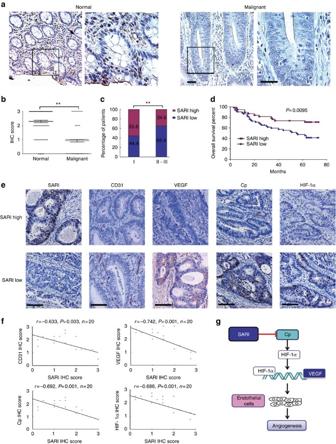Figure 7: Validation of SARI in human colon cancer tissue microarray. (a) Analysis of tissue microarrays (TMAs). Staining for SARI on TMAs containing 135 normal and malignant colon tissues. Scale bar, 100 μm. (b) Statistical analysis was performed using the GraphPad Prism 5 program to compare the relative levels of SARI between normal and malignant colon tissues (Mann–Whitney test;n=135; **P<0.01; Student’st-test). Black triangles indicate the colon sample, and the transverse lines indicate the mean. (c) Percentage of patients with high and low expression of SARI according to tumour differentiation stage. Numbers in bars represent the percentage of patients. (n=90; **P<0.01; Student’st-test). (d) Kaplan–Meier curve showing overall survival of patients (in percentage) with colon cancer, stratified by SARI expression (high- and low-scoring tumours). SARI expression was determined by immunohistochemistry staining and scored as described in methods. The log-rank test was used to compare differences between groups (n=90;P=0.0095; long-rank test). (e,f) Correlation analyses of SARI, VEGF, Cp and CD31 in of human malignant colon tissues from 20 patients. SARI, VEGF, CD31, Cp and HIF-1α expression levels were determined by immunohistochemistry staining and scored as described in methods (e). Scale bar, 100 μm. Pearson’s correlation coefficient (r) andPvalue are shown (f;n=20; Pearson analysis). (g) Model for angiogenesis inhibition by SARI through direct targeting of Cp and subsequent inactivation of the HIF-1α/VEGF axis. Figure 7: Validation of SARI in human colon cancer tissue microarray. ( a ) Analysis of tissue microarrays (TMAs). Staining for SARI on TMAs containing 135 normal and malignant colon tissues. Scale bar, 100 μm. ( b ) Statistical analysis was performed using the GraphPad Prism 5 program to compare the relative levels of SARI between normal and malignant colon tissues (Mann–Whitney test; n =135; ** P <0.01; Student’s t -test). Black triangles indicate the colon sample, and the transverse lines indicate the mean. ( c ) Percentage of patients with high and low expression of SARI according to tumour differentiation stage. Numbers in bars represent the percentage of patients. ( n =90; ** P <0.01; Student’s t -test). ( d ) Kaplan–Meier curve showing overall survival of patients (in percentage) with colon cancer, stratified by SARI expression (high- and low-scoring tumours). SARI expression was determined by immunohistochemistry staining and scored as described in methods. The log-rank test was used to compare differences between groups ( n =90; P =0.0095; long-rank test). ( e , f ) Correlation analyses of SARI, VEGF, Cp and CD31 in of human malignant colon tissues from 20 patients. SARI, VEGF, CD31, Cp and HIF-1α expression levels were determined by immunohistochemistry staining and scored as described in methods ( e ). Scale bar, 100 μm. Pearson’s correlation coefficient ( r ) and P value are shown ( f ; n =20; Pearson analysis). ( g ) Model for angiogenesis inhibition by SARI through direct targeting of Cp and subsequent inactivation of the HIF-1α/VEGF axis. Full size image Prior studies have shown that SARI has a broad expression profile, but is not expressed in most malignant tissues [15] . However, the expression of SARI in colon cancer cell lines or normal/malignant colon tissues from patients, let alone the role of SARI in colon tumour formation, was still unclear. Our study demonstrated that SARI is downregulated in most colon cancer cell lines, except in HCT15 and SW620 cancer cells at the mRNA and protein levels. Furthermore, TMA staining was performed and found that compared with normal colon tissues, SARI expression was significantly reduced in 106 (78.52%) of 135 malignant colon cancer specimens. Taken together, these results indicate that SARI is downregulated in most colon cancer cell lines and malignant cancer specimens from patients. The AOM/DSS-induced colonic tumorigenesis model is a standard and widely used model for simulating colonic tumour formation and progression [21] , [22] . In this study, SARI −/− and SARI WT mice were used in the AOM/DSS-induced colonic tumorigenesis model, and our results first indicated that more colonic tumour was found in the SARI −/− mice after AOM/DSS treatment. Thus, we hypothesized that SARI is an inhibitor of colonic tumour formation. To address this hypothesis further, colon cancer cells with stable SARI expression were selected, and the subsequent subcutaneous mouse model results demonstrated that overexpression of SARI in SW480 and HCT116 cells significantly inhibited tumour growth. Moreover, knockdown of SARI in HCT15 cells by shSARI-1068 or shSARI-554 significantly promoted HCT15 subcutaneous tumour growth. Collectively, our data suggest that SARI functions as a tumour suppressor. Tumour growth is a complicated biological process, and blood vessels are necessary for supplying nutrients and oxygen to the tumour [23] . Thus, anti-angiogenesis strategies are often effective for cancer therapy [24] , [25] . In this study, we demonstrated a novel function of SARI in inhibiting angiogenesis in colon tumour growth. Angiogenesis was significantly inhibited by SARI in SW480 and HCT116 subcutaneous tumours, and more angiogenesis was observed in the HCT15 subcutaneous tumour after knockdown of SARI. More importantly, SARI deficiency induces angiogenesis in AOM/DSS-induced colonic tumours. HUVEC-related and Matrigel plug assays were employed to demonstrate that SARI is a novel inhibitor of angiogenesis. After inhibition of angiogenesis, more necrotic and hypoxic areas were observed in the SW480-SARI and HCT116-SARI tumours. Further analysis indicated that there is an inverse and close correction between angiogenesis and apoptosis in subcutaneous tumours. We have reason to believe that angiogenesis contributes to the SARI-regulated colon tumour growth. Angiogenesis is regulated by the balance of various proangiogenic stimulators and angiogenesis inhibitors [26] , [27] .To assess the target of SARI on the inhibition of angiogenesis, an angiogenesis antibody array was performed and indicated that several pro-angiogenesis cytokines were downregulated by SARI, including VEGF, PLGF, EGF, bFGF and PDGF-BB. In addition, ELISA, western blotting, real-time PCR and immunostaining showed that VEGF is significantly reduced by SARI in both SW480 and HCT116 colon cancer cells. Furthermore, shRNA-targeting VEGF and HUVEC-related assays were performed to demonstrate that VEGF plays a central role in SARI-inhibited angiogenesis. VEGF is a potent angiogenic molecule, as well as a prime molecule responsible for tumour progression and metastasis by enhancing angiogenesis [28] , [29] . Thus, VEGF is a frequent target for therapy. Several VEGF-targeted therapies have shown promise [25] , [30] , [31] , especially Bevacizumab (Avastin), a humanized monoclonal antibody of VEGF widely used in the treatment of various cancers and other diseases. According to the significant effects of SARI on reducing VEGF expression observed in vivo and in vitro , SARI may be a potential target for targeted therapy. VEGF expression is regulated by several pathways and transcriptional factors at the translation or transcriptional level [32] . To determine the direct target of SARI in the regulation of VEGF expression, we employed Co-IP/SDS–PAGE, followed by MS analysis. Co-IP, immunofluorescence and western blotting demonstrated that Cp was the direct target of SARI. Cp is a ferroxidase important in the regulation of both systemic and intracellular iron levels [33] . Inhibition of Cp has been demonstrated to suppress tumour growth and angiogenesis in breast cancer [34] . In our study, we found that Cp expression was markedly inhibited by SARI in the nucleus under normoxia and hypoxia via a protease degradation pathway. The kinetic analysis of Cp protein degradation indicated that Cp protein degraded faster in the SARI cells than in the control cells. Cp plays an important role in the stabilization and nuclear transport of HIF-1α, thus regulating VEGF expression [20] . Meanwhile, Cp being a well-established HIF-1α target gene, one would expect that hypoxia would stabilize HIF-1α and upregulate Cp again in a self-feeding feedback loop [35] , [36] . In line with the reduction of Cp, HIF-1α expression was found to be inhibited by SARI. Further results demonstrated that knockdown or overexpression of Cp blocks the regulation of SARI on HIF-1α and VEGF expression, and angiogenesis under normoxic and hypoxic conditions. In addition, inhibition of HIF-1α also blocks the regulation of SARI on Cp and VEGF expression, and angiogenesis under normoxic and hypoxic conditions. It was indicated that SARI inhibits the Cp-HIF-1α self-feeding feedback loop and the activity of the HIF-1α/VEGF axis through directly targeting Cp. Moreover, in colonic tumours from AOM/DSS-induced tumorigenic mice, increased angiogenesis and expression of Cp, HIF-1α and VEGF was observed in those with the SARI knockout. This is consistent with the results seen in colon cancer cell lines and xenograft tumours. According to the above results, a mechanistic model of SARI in the inhibition of angiogenesis was established ( Fig. 7g ). This model lays foundation for understanding the mechanism and effects of SARI on angiogenesis. It has been demonstrated that mutation of leucine into proline 59 in the bZIP domain of SARI completely inhibits interaction between c-Jun and SARI [15] , indicating that the leucine zipper motif mediates this interaction. It should be noted that the foundation of the carboxyterminal domain of SARI (from 80 to 274 amino acids of SARI) is still elusive. Our study first demonstrated that the binding site of Cp is localized among amino acids 80–274 of SARI, but the exact binding site should be determined in the further studies. Prior studies have demonstrated that SARI expression inversely correlates with poor prognosis of patients with hepatocellular carcinoma and oral tongue squamous cell cancer [37] , [38] . The recent study by Liu et al . demonstrated that SARI deficiency promotes CRC progression and correlates with a worse patient prognosis [19] . In this study, we also found that SARI expression inversely correlates with tumour stage and the poor prognosis of patients with colon cancer. Furthermore, for the first time, we detected a significant inverse correction between the expression of SARI and CD31, SARI and VEGF, SARI and Cp, and SARI and HIF-1α. These observations are consistent with the role of SARI in the downregulation of Cp, HIF-1α and VEGF, and the inhibition of angiogenesis in tumour bearing HCT116 and SW480 xenograft tumours and AOM/DSS-induced colonic tumour. Since HIF-1α and VEGF expression and angiogenesis in tumours correlate with poor prognosis of patients with cancer [28] , [29] , [39] , [40] , [41] , it indicates that SARI expression inversely correlates with poor prognosis of patients with colon cancer. Collectively, these findings indicate that SARI may be a novel potential biomarker for the prognosis of patients with colon cancer. In summary, we first demonstrate that SARI inhibits angiogenesis by directly targeting Cp and inhibiting the HIF-1α/VEGF axis with important implications for colon tumour formation in AOM/DSS-induced colonic tumorigenesis and colon cancer cell subcutaneous cancer models. Moreover, we provide TMA evidence that SARI expression inversely correlates with advanced stage and positively correlates with the survival of patients with colon cancer. Collectively, our study suggests that SARI may be an effective indicator for prognosis and a potential target for colon cancer therapy, and perhaps other cancers. Cell lines and antibodies All colon cancer cell lines (Caco-2, Lovo, SW480, HCT116, DLD-1, HT29, SW620, HCT15 and SW837) were purchased from American Type Culture Collection (ATCC, Manassas, VA, USA) and cultured in DMEM supplemented with 10% fetal bovine serum (FBS) and antibiotics. Cell line authentication was assessed using a short tandem repeat DNA profiling method in our laboratory, and the latest verification was done in July 2013. The mycoplasma detecting kit (catalogue no. MD001), purchased from Shanghai Yise Medical Technology was performed to test whether there are mycoplasma contamination in all cells. HUVECs were maintained as described previously [42] and cultured in EndoGRO-VEGF medium (Millipore, MA, USA). Antibodies used in this study were as follows: SARI (ab157466, Abcam, London, UK), SARI (241887, Santa Cruz Biotechnology, Santa Cruz, CA, USA), SARI (Zhengneng bio, Chengdu, China, for detecting mouse SARI protein), Cp (ab48614, Abcam), HIF-1α (H6536, Sigma, MO, USA), HA (04–902, Millipore), VEGF (ab46154, Abcam), CD31 (550274, BD Biosciences, CA, USA), CD31 (ZM-0044, ZSBIO, Beijing, China, for detecting human CD31), Histone H3 (4499P, CST, MA, USA), GAPDH (sc365062, Santa Cruz Biotechnology) and β-actin (sc-47778, Santa Cruz Biotechnology). Mice Female BALB/c nude mice were purchased from the Model Animal Research Center of Nanjing University (Nanjing, China) and allowed to acclimate for 1 week before use. The SARI knockout (SARI −/− , catalogue no. 019085) and SARI wild-type (SARI WT , catalogue no. 002448) mice were purchased from the Jackson Laboratory ( http://jaxmice.jax.org/strain/019085.html ). All mouse care and experiments were carried out in accordance with institutional guidelines concerning animal use and care of Sichuan University. Mouse gene type was determined according to the genotyping protocols supplied by the Jackson Laboratory ( http://jaxmice.jax.org/strain/019085.html ). AOM/DSS-induced colonic tumorigenesis model AOM and DSS were purchased from Sigma and MP Biomedicals, separately. The model used was established in a previous study [22] . In brief, 10 mg AOM/Kg mouse body was injected into the peritoneal of mice on the first day. After 7 days, 2% DSS was added into the drinking water for the mice and maintained for 7 days, and then removed for 14 days intervals. Four cycles of DSS are needed to establish this model. After 98 days, the mice were killed and used for subsequent experimentation. The tumour numbers per colon were counted as previous described [22] . The average tumour diameter was measured with the help of a sliding caliper as previous described [22] . Tumour size was calculated as length × width (mm 2 ). The total surface area of tumours per colon was analysed among the different groups. Enzyme-linked immunosorbent assay The supernatant from the cancer cells was collected, and the cell number was counted by a Scepter 2.0 (Millipore). The supernatant was used to measure the total levels of several cytokines using the human VEGF ELISA kit (NeoBioscience, Shenzhen, China), PDGF-BB ELISA kit (Boster, Wuhan, China), bFGF ELISA kit (NeoBioscience), VEGF-C ELISA kit (Boster), PIGF ELISA kit (NeoBioscience) and VEGF-D ELISA kit (NeoBioscience) according to the manufacturer’s instructions. The cytokine expression level (pg ml −1 ) per 10 5 cancer cells was analysed. Human angiogenesis antibody array The human angiogenesis antibody array kit was purchased from RayBiotech (AAH-ANG-1-8, Norcross, GA). A total of 2 × 10 5 control and SARI cells were plated in the well of a six-well plate with 2 ml of DMEM medium containing 10% FBS. And 48 h later, the conditioned medium was collected and used for human angiogenesis antibody array analysis. The procedure followed the manufacturer’s instructions. In brief, the angiogenesis antibody membranes were placed in a four-well multi-dish with 2 ml of array blocking buffer. The membrane was incubated for 30 min on a rocking platform. After the incubation, the blocking buffer was removed, the antibody membrane was washed twice with the array wash buffer and 1.5 ml of conditioned medium was added into the well. The membrane was incubated for 3 h at room temperature on an orbital shaker, and then washed with array wash buffer I and II twice. Then, 1 ml of streptavidin-horseradish peroxidase solution was added onto the membrane and incubated for 2 h at room temperature on an orbital shaker. Next, three washes were performed with array wash buffer I and II twice. A chemiluminescent substrate ECL kit supplied in the kit was used to take detailed pictures of the array. Image J software was used to quantify the arrays. Matrigel plug assay BALB/c nude mice (6 weeks of age) were given subcutaneous injections of 500 μl of Matrigel (BD Biosciences) containing 1 × 10 6 cancer cells at 4 °C. Seven days later, the plug was fixed and stained for CD31(1:200, BD biosciences) and VEGF(1:100, Millipore). RNA interference The lentivirus-based expression vectors containing the SARI or negative control (NC) siRNA were provided by GenePharma (Shanghai, China). The lenti-shRNA and lenti-shNC were used to infect colon cancer cells to knockout SARI. The plasmid-based expression vectors containing the VEGF of NC siRNA were also provided by GenePharma. The p-shVEGF and p-shNC were used to transfect colon cancer cells to knockout VEGF. The effective siRNA sequence was identified and used in subsequent experiments. The tetracycline-regulated expression system The tetracycline-regulated system was supplied by Biowit Tech (Shenzhen, Guangdong, China). The Tet-SARI and Tet-control plasmid were exacted and used to transfect SW480 cells. The protein lysis and conditional medium were collected for analysis by western blot and ELISA. VEGF-trap treatment and VEGF recovery VEGF protein and VEGF-trap antibody were purchased from R&D Systems (MN, USA) and Bayer (Leverkusen, Germany) separately. VEGF-neutralizing antibody (VEGF-Trap) was added into the conditional medium of control and SARI cells at a concentration of 400 nM, as previous studies in our laboratory indicated this concentration as optimal [43] . The VEGF protein was added into the conditioned medium of SARI cells to recover the VEGF concentration to that of the conditioned medium of the control cells. Subcellular protein extraction A subcellular protein extraction kit (Millipore) was employed to extract cytosolic and nuclear proteins. The procedure was performed according to the kit instructions. Histone H3 was used as the nuclear protein loading control and β-actin was used as the cytosolic protein loading control. RT–PCR and real-time PCR Total RNA was extracted from cells using TRIzol reagent (Invitrogen, Carlsbad, CA, USA). RNA samples (1 μg) were subjected to RT–PCR using the TaKaRa One-step RT-PCR kit (Takara, Shiga, Japan). All PCR products were separated by electrophoresis in 1% agarose gels and were visualized using GoldView. For real-time PCR, resulting complementary DNA was analysed in triplicate using SYBR Green (Takara). Relative mRNA concentrations were determined by 2 −ΔΔCt , where Ct is the mean threshold cycle difference after normalization to U6 values. Western blotting After inhibitor treatment or plasmid transfection, the control and SARI cells were collected and lysed on ice for 30 min with the RIPA lysis buffer (Beyotime, Nanjing, China) containing 1% protease inhibitor cocktail (Merck Millipore). The lysis was centrifuged for 15 min by 12,000 g at 4 °C, and the supernatants were collected. The Bradford protein assay kit (Thermo Scientific, MA, USA) was employed to determine the protein concentrations. An amount of 20 μg protein with equal amount was loaded and separated by SDS–PAGE gel electrophoresis, followed by the transfer of proteins onto the polyvinylidenedi fluoride membranes (Merck Millipore). After blocking with TBS/T buffer containing 5% milk, the membranes were incubated with the primary antibodies against SARI (1:400, Abcam), Cp (1:1500, Abcam), HIF-1α (1:800, Abcam), GAPDH (1:50,000, CST) and VEGF (1:1,000, Millipore) in 5% milk TBS/T buffer overnight at 4 °C. Following incubation with horseradish peroxidase-conjugated secondary antibodies (Zsbio, Beijing, China) at room temperature for 1 h, the bands were detected using a chemiluminescent substrate ECL kit (Merck Millipore). Immunofluorescence analysis A total of 2 × 10 4 control and SARI cells were plated in EZ-slide (Merck Millipore) with 0.5 ml DMEM medium containing 10% FBS. Twenty-four hours later, 4% paraformaldehyde was employed to fix the cells at room temperature for 10 min. Then, the cells were blocked with goat serum and incubated with primary antibodies against SARI (1:200, Abcam; 1:100, Santa Cruz, TX, USA), VEGF (1:200, Millipore) and Cp (1:400, Abcam) for 1.5 h at 37 °C, followed directly by either fluorescein isothiocyanate (FITC) or Texas Red-conjugated secondary antibodies (1:200, Santa Cruz) for 1.5 h at 37 °C. Nuclei were counterstained with DAPI (Roche, Basel, Switzerland). All specimens were evaluated using an Olympus BX600 microscope and SPOT Flex camera. In vitro tube formation and invasion assay A total of 2 × 10 5 control and SARI cells were plated in the well of a six-well plate with 2 ml of DMEM medium containing 10% FBS. And 48 h later, the conditioned medium was collected and used for in vitro tube formation and invasion assay. For the tube formation assay, the wells of a 96-well plate were coated with 50 μl ice-cold BD Matrigel (BD Biosciences). HUVECs (20,000) in 100 μl of conditioned medium were added into the well that plated with Matrigel. HUVECs were incubated for 4–6 h at 37 °C and then visualized by light microscopy. The amount of branch points (≥3 cells per branch) were counted and analysed in five random fields per replicate. For the invasion assay, diluted Matrigel (1:6 dilution with blank medium) was added into the cell culture inserts (8 μm, 24-well format, Millipore). And 30 min later, HUVEC (10,000) in 200 μl of conditioned medium were added to the upper chamber, while the lower chamber was filled with 1 ml of conditioned medium. The culture was maintained for 72 h. Then, the cell culture inserts were collected and the cells on the upper side of the filters were removed with cotton-tipped swabs. The cells on the underside of the filters were fixed with 4% formaldehyde for 10 min and stained with crystal violet for 10 min. The stained cells were counted in five randomly chosen fields. And the results are presented as the number of invasive cells in per field. Hypoxia assays Hypoxyprobe-1-Mab1 (Hypoxyprobe kit) was purchased from the Chemicon (MA, USA) and used for detecting the hypoxia area in tumours, following the manufacturer’s instructions. Pimonidazole hydrochloride compound was intraperitoneal injected into tumour-bearing mice. After injection for 1 h, the mice was killed and the subcutaneous tumour sections were immunostained to detect pimonidazole adducts by adding FITC-labelled Mab1 and incubating for 2 h. Nuclei were detected with DAPI. All specimens were evaluated using an Olympus BX600 microscope and SPOT Flex camera. Immunostaining and histology Frozen or paraffin sections were used for immunohistochemical analysis. Vessel imaging on frozen sections was performed by staining with a 1:400 dilution of a rat anti-mouse CD31 antibody (BD Biosciences). SARI and control tumours were frozen and stained with SARI (1:200, Abcam), VEGF (1:200, Abcam), HIF-1α (1:400, Abcam) and dually immunostained for cleaved caspase-3 (1:100, CST) and CD31 (1:400, BD biosciences). For fluorescent visualization of antibody reactions, secondary antibodies were labelled with the FITC-Texas Red, while the nuclei were detected with DAPI. All specimens were evaluated using an Olympus BX600 microscope and SPOT Flex camera. Tumours were scored by counting the number of cancer cells expressing the proteins as determined by SARI, VEGF and CD31 staining in tumours. The number of cleaved caspase-3-positive cells and vessel number were both counted per mm 2 and the correlation was analysed. Tissue microarray The cohort of 135 pairs of human malignant colon cancer tissues and their corresponding adjacent noncancerous colon tissues was purchased from Shanghai Outdo Biotech. Co. Ltd (Shanghai, China) and approved by the Ethics Committee of Taizhou Hospital. Colon cancer patients (age from 55 to 75 years old; clinical tumour grade from II-A to III-B) were recruited for biopsy at the West China Hospital (Chengdu, China) and approved by the Ethics Committee of West China Hospital. The tissue was fixed with 4% paraformaldehyde and the sections were used to determine SARI, CD31, VEGF, Cp and HIF-1α expression by immunohistochemistry. Tumours were scored by counting the number of cancer cells expressing the proteins as determined by SARI, VEGF, Cp, HIF-1α and CD31 staining in tumours. The correlation between SARI, CD31, VEGF, Cp and HIF-1α expression in human colon cancer tissue was analysed based on the immunohistochemistry (IHC) score. Animal studies Studies were performed in accordance with institutional guidelines concerning animal use and care. HCT116 and SW480 cells (5 × 10 6 cells) stably expressing SARI or control and HCT15-shNC, and shSARI-1068 and shSARI-554 cells (2 × 10 6 cells) were injected into the flank of female BALB/c nude mice to establish a subcutaneous cancer model. Tumour size was determined by collecting length and width measurements, and calculating the tumour volume (mm 3 ) as (tumour length × (tumour width) 2 ) × 0.52. When mice were killed, tumours from each animal were collected, weighed and used for histopathological studies. Statistical analysis All experiments were repeated three to five times, and the data were expressed as the mean±s.d. Statistical analysis was performed by the Student’s t -tests for comparing two groups and by analysis of variance for multiple group comparisons; P <0.05 was considered statistically significant. Kaplan–Meier curves and the log-rank test were used to compare survival times among the groups. The Pearson correlation analysis was performed to determine the correlation among the groups. All calculations were performed using SPSS v17.0 (SPSS Inc., Chicago, IL, USA). Data availability Data supporting the findings of this study are available within the article and its Supplementary Information Files and from the corresponding author upon reasonable request. How to cite this article: Dai, L. et al . SARI inhibits angiogenesis and tumour growth of human colon cancer through directly targeting ceruloplasmin. Nat. Commun. 7:11996 doi: 10.1038/ncomms11996 (2016).